Diverse and divergent protein post-translational modifications in two growth stages of a natural microbial community Detailed characterization of post-translational modifications (PTMs) of proteins in microbial communities remains a significant challenge. Here we directly identify and quantify a broad range of PTMs (hydroxylation, methylation, citrullination, acetylation, phosphorylation, methylthiolation, S-nitrosylation and nitration) in a natural microbial community from an acid mine drainage site. Approximately 29% of the identified proteins of the dominant Leptospirillum group II bacteria are modified, and 43% of modified proteins carry multiple PTM types. Most PTM events, except S-nitrosylations, have low fractional occupancy. Notably, PTM events are detected on Cas proteins involved in antiviral defense, an aspect of Cas biochemistry not considered previously. Further, Cas PTM profiles from Leptospirillum group II differ in early versus mature biofilms. PTM patterns are divergent on orthologues of two closely related, but ecologically differentiated, Leptospirillum group II bacteria. Our results highlight the prevalence and dynamics of PTMs of proteins, with potential significance for ecological adaptation and microbial evolution. Microbial communities populate and shape diverse ecological niches within natural environments [1] . The physiology of organisms in natural consortia and their responses to changing environmental conditions have been studied by measuring the abundance changes of proteins across a series of field samples using community proteomics [2] , [3] , [4] . However, microorganisms in a community regulate their metabolic processes not only by changing the copy numbers of proteins, but also by modulating the specific activities of expressed protein molecules. Post-translational modifications (PTMs) are one of the most important mechanisms for activating, changing or suppressing proteins’ functions [5] . Phosphorylation cascades are the mechanisms for many signal transductions, such as two-component systems [6] and cell-division cycle control [7] . Acetylation preferentially targets large protein complexes and regulates key metabolic pathways [8] , including glycolysis and gluconeogenesis in bacteria [9] . Proteome-wide interactions between phosphorylation and acetylation have been observed in the bacterium Mycoplasma pneumoniae [10] . Methylation is actively involved in mediating protein–protein interactions through methylation-dependent binding domains [11] . Phosphorylation and methylation were found to collectively regulate signalling during bacterial chemotaxis [6] . S-nitrosylation and nitration, caused by reactive nitrogen species, are the major signalling mechanisms under nitrosative and oxidative stress [12] , [13] . Citrullination of arginine plays critical roles in regulation of gene expression by changing DNA–protein interaction [14] . Hydroxylation has been primarily found in collagen [15] and beta-methylthiolation has been mainly observed in bacterial ribosomal proteins [16] , but their scope and significance in various complex biological processes remain unclear. Because of the functional roles of PTMs in regulating biological activities, PTMs may be conserved across orthologous proteins, and the divergence of PTMs may contribute to phenotypic diversity [17] . Recently, phosphorylation, acetylation and ubiquitination were compared between different eukaryotic species, and divergent PTM patterns were revealed between their orthologues [18] , [19] , [20] , [21] , [22] . However, the conservation of PTMs in bacteria and archaea is largely unknown. The UBA and 5wayCG variants of Leptospirillum group II, typically dominating acid mine drainage (AMD) biofilms [23] , have been shown to exhibit substantial ecological differentiation [24] . These Nitrospirae phylum bacteria with 99.7% 16S rRNA gene sequence identity exist as a continuum of genotypes that have undergone varying degrees of recent large-scale homologous recombination [25] and, therefore, are ideal for studying the PTM conservation between closely related, co-evolving microorganisms. PTMs can be identified using a shotgun proteomics approach by searching for modified peptides in liquid chromatography-tandem mass spectrometry (LC-MS/MS) data. Previous in-depth PTM studies have generally targeted specific types of PTMs by enriching modified peptides via affinity purification before LC-MS/MS analysis. Although enrichment reduces the sample complexity, the measurements do not provide a comprehensive PTM profile of proteins that may carry many types of PTMs unless a separate enrichment is used for each PTM type [26] , [27] . Furthermore, enrichment does not permit direct quantification of PTM fractional occupancy, which is the percentage of the copies of a protein that is modified with a specific PTM event [28] , [29] . Here, to overcome the limitations of enrichment-based approaches, we use an optimized global shotgun proteomics approach for broad-range PTM identification and quantification. The eight types of PTMs described above are simultaneously measured in two samples of a natural microbial biofilm community growing in an AMD environment. The proteomic PTM profiles are compared between two biofilm growth stages to uncover the dynamics of PTMs during community succession. We find divergent PTM patterns on many orthologous proteins of Leptospirillum group II bacteria, further underlining metabolic distinction of these closely related organisms [24] . Identification of diverse PTMs in microbial community proteomes Large intact sheets of AMD biofilm were sampled at the AB Muck Dam site in the Richmond Mine at Iron Mountain, CA, on 17 September 2010 (pH ~1, 39 °C). Two samples were collected only centimeters apart: a thin, early growth-stage biofilm community (GS1), and a late growth-stage biofilm community represented by a thicker portion of the biofilm (GS2) ( Fig. 1 ). 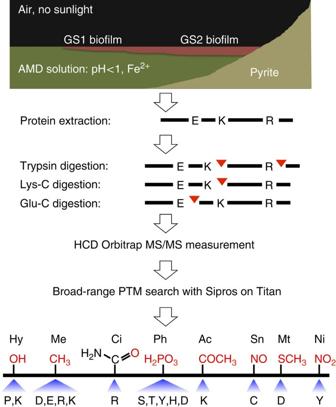Figure 1: Study overview. AMD biofilms representing two growth stages (GS1 and GS2) were collected from a site within the Richmond Mind. Proteome samples were digested using three proteases in parallel and analysed by HCD MS/MS. The following biological PTMs were searched: hydroxylation (Hy), methylation (Me), citrullination (Ci), phosphorylation (Ph), acetylation (Ac), S-nitrosylation (Sn), methylthiolation (Mt) and nitration (Ni). The chemical formula (red) and modifiable amino acids are listed for each type of PTM. Figure 1: Study overview. AMD biofilms representing two growth stages (GS1 and GS2) were collected from a site within the Richmond Mind. Proteome samples were digested using three proteases in parallel and analysed by HCD MS/MS. The following biological PTMs were searched: hydroxylation (Hy), methylation (Me), citrullination (Ci), phosphorylation (Ph), acetylation (Ac), S-nitrosylation (Sn), methylthiolation (Mt) and nitration (Ni). The chemical formula (red) and modifiable amino acids are listed for each type of PTM. Full size image Three protein samples were prepared in parallel for each AMD biofilm sample, digested with trypsin, Lys-C or Glu-C. Each protein digest sample was analysed in technical duplicate by 22-hour LC-MS/MS using an LTQ Orbitrap Elite mass spectrometer. We optimized the high-resolution MS/MS method using higher-energy collisional dissociation (HCD) [30] . Spectral quality and identification results were significantly improved by using the mass-to-charge ratio ( m / z ) cutoff of 180 in MS/MS scans, normalized collision energy of 30% for HCD and minimum ion threshold of 1,000 for MS/MS triggering. We compared the optimized high-resolution MS/MS method with a conventional low-resolution MS/MS method based on collision-induced dissociation (CID) using a test AMD biofilm sample. The two methods identified comparable numbers of peptide-spectrum matches (PSMs) and peptides ( Supplementary Table 1 ). However, the high-resolution MS/MS method identified 71% of the acquired fragment ion spectra and provided high mass accuracy (<0.01 Da mass error) on matched fragment ions, which allowed searching a much larger sequence space with a low false discovery rate (FDR). In addition to the eight biological PTMs described above (hydroxylation, methylation, citrullination, acetylation, phosphorylation, methylthiolation, S-nitrosylation and nitration), we also searched for three PTMs commonly resulting from proteome sample preparation, including oxidation of methionine, deamidation of asparagine and glutamine and alkylation of cysteine. Because simultaneous consideration of these types of PTMs vastly expanded the sequence space for database searching, the database searching was performed with a scalable Sipros [31] , [32] algorithm on a supercomputer, Titan, using up to 35,000 central processing unit cores across 1,000s of compute nodes. Identification results were organized in a hierarchical structure with five levels: organisms, proteins or protein groups, PTM events, peptides and PSMs. An identification at a given level generally comprised multiple identifications at the next lower level. A PTM event was defined as a specific type of PTM on a specific residue of a protein. As identification results were pooled across trypsin, Lys-C and Glu-C digests of a sample, many PTM events were covered by multiple peptides. We identified 765,202 and 743,413 PSMs, 78,539 and 104,893 non-redundant peptides, 3,599 and 3,723 unique PTM events and 4,259 and 5,055 proteins or protein groups from seven major organisms in the GS1 and GS2 biofilm, respectively ( Table 1 and Supplementary Data 1 and 2 ). Consistent with previous observations [33] , the GS1 biofilm had low diversity and was comprised predominantly of Leptospirillum bacteria, whereas the GS2 biofilm harboured a more diverse community with increased abundance of archaeal species, as indicated by proteomics results. Approximately 76% of the PSMs and 46% of the unique PTM events were identified from the UBA or 5wayCG Leptospirilli . The FDR, estimated by searching concatenated reverse sequences [34] , was ~0.34% at the PSM level, ~1.0% at the peptide level, ~2.0% at the PTM event level and ~3.5% at the protein or protein group level. The FDRs in the identification hierarchy increased because upper-level identifications from reverse sequences often comprised far fewer lower-level identifications than those from forward sequences. Adding longer Lys-C and Glu-C peptides to tryptic peptides nearly tripled the number of identified PTM events. Table 1 Summary of identification results at the PSM, peptide, PTM event, and protein or protein group levels. Full size table The PTM events identified from the GS1 and GS2 samples were categorized by PTM types and organisms ( Fig. 2 ). Because of the ~95% average amino acid identity between orthologous proteins of the UBA and 5wayCG Leptospirilli , ~2,700 PTM events unique to the Leptospirillum group II cannot be resolved to a specific organism (shared Lepto II, Fig. 2 ). Hydroxylation, methylation and citrullination were the most commonly identified PTM types. In the Leptospirillum group II proteomes, ~29% of the identified proteins were modified with at least one unique PTM event in a biofilm sample. Of these modified proteins, ~43% carried multiple types of unique PTM events. Some extensively modified proteins included chaperone proteins, such as DnaK, GroEL and ClpB, enzymes in the reductive tricarboxylic acid (rTCA) cycle, and proteins involved in iron oxidation and electron transport, such as NADH dehydrogenase and several cytochromes. 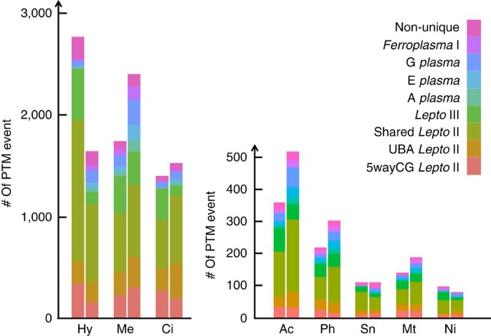Figure 2: Histograms of identified PTM events in the AMD community. For each PTM type, the numbers of PTM events were compared among major community members (colour-coded sections) between GS1 (left bar) and GS2 (right bar). SharedLeptospirillum(Lepto) group II represents PTM events that can be only assigned to theLeptospirillumgroup II, but cannot be resolved to a specific organism. Ac, acetylation; Ci, citrullination; Hy, hydroxylation; Me, methylation; Mt, methylthiolation; Ni, nitration; Ph, phosphorylation; Sn, S-nitrosylation. Figure 2: Histograms of identified PTM events in the AMD community. For each PTM type, the numbers of PTM events were compared among major community members (colour-coded sections) between GS1 (left bar) and GS2 (right bar). Shared Leptospirillum ( Lepto ) group II represents PTM events that can be only assigned to the Leptospirillum group II, but cannot be resolved to a specific organism. Ac, acetylation; Ci, citrullination; Hy, hydroxylation; Me, methylation; Mt, methylthiolation; Ni, nitration; Ph, phosphorylation; Sn, S-nitrosylation. Full size image Because confident identification of a PTM event requires placement of that PTM on the correct residue, we separately estimated the accuracy of PTM localization by re-analyzing the HCD high-resolution MS/MS data of synthetic peptides with known phosphorylation sites from a recently published study [35] . The phosphorylation events were assigned to the correct residues for more than 97% of the modified spectra with PTM localization (that is, DeltaP >0 for site differentiation) by Sipros ( Supplementary Data 3 ). We then evaluated the depth and breadth of our broad-range PTM identification approach with a model organism, Escherichia coli . A total of 5,005 unique PTM events were found from 966 proteins out of a total of 2,082 identified proteins ( Supplementary Table 2 and Supplementary Data 1 and 2 ). Hydroxylation, citrullination and methylation were the three most abundant PTM types in laboratory-grown E. coli , which was consistent with the results of the AMD microbial communities. Previous enrichment-based measurements identified ~150 phosphorylation events [36] and ~1,070 acetylation events [37] in E. coli . Here, our approach simultaneously identified 284 unique phosphorylation events and 470 unique acetylation events. Although the PTM identification results were not directly comparable between different E. coli samples used in these measurements, our approach was successful in finding extensive modifications of proteins by many different types of PTMs without using multiple enrichments. For example, the transcriptional factor OxyR was recently discovered as a master regulator of S-nitrosylation in E. coli under anaerobic respiration on nitrate [12] . Here, we identified 176 unique S-nitrosylation events from 159 proteins under aerobic growth condition, including OxyR. In addition to the S-nitrosylation, OxyR was simultaneously modified with phosphorylation, methylation and acetylation. PTM dynamics of the community during ecological succession We compared the unique and localized PTM events in UBA and 5wayCG Leptospirilli between the GS1 and GS2 samples. Although ~75% of the proteins were identified in both samples, only ~17% of the organism-specific PTMs were maintained between the two samples ( Fig. 3 and Supplementary Figs 1 and 2 ). PTMs that differed between samples were significantly enriched ( P -value <0.05, two-tailed Fisher’s exact test) in citrullination and methylation. These PTMs may be involved in regulation of pathway activities. For instance, Leptospirillum group II was previously found to have different chemotaxis and motility activities between the two growth stages, possibly reflecting the diversified community membership and increased competition for nutrients in GS2 (ref. 38 ). The PTM patterns were compared between GS1 and GS2 for the chemotaxis gene clusters in the Leptospirillum group II and III ( Fig. 4a,b ) [39] . While all proteins from the two gene clusters were identified, they had distinct PTM patterns in the two growth stages. More methylation events were identified in GS2 than in GS1 on the chemotaxis scaffolding protein CheW (locus ID: CGL2_11277G0245 and UBAL2_8241G0195, where CGL2 and UBAL2 denote 5wayCG- and UBA-type orthologues, respectively), histidine kinase CheA (CGL2_11277G0248 and UBAL2_8241G0198), response regulator CheY (CGL2_11277G0249 and UBAL2_8241G0199), and methyl-accepting chemotaxis protein MCP (CGL2_11277G0246 and UBAL2_8241G0196) from Leptospirillum group II and on the CheY (UBAL3_8063G0048) and flagellar sigma factor FliA (UBAL3_8063G0049) from Leptospirillum group III. Citrullination was extensively found across many proteins. A cluster of hydroxylation events was only identified on the Leptospirillum group II MCP in GS1. Two phosphorylation events were identified on the motility protein A MotA (CGL2_11277G0244 and UBAL2_8241G0194) and chemotaxis methylesterase CheB (CGL2_11277G0247 and UBAL2_8241G0197) from Leptospirillum group II only in GS2. An acetylation event was identified on the motility protein B (MotB; UBAL3_8063G0043) from Leptospirillum group III in GS1. 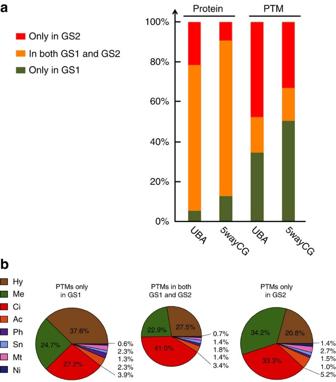Figure 3: Dynamics of proteins and organism-specific PTM events between the two growth stages in the UBA and 5wayCGLeptospirilli. (a) The percentages of proteins and PTM events identified only in GS1 (green sections), in both GS1 and GS2 (orange sections), and only in GS2 (red sections). (b) The distribution of organism-specific PTM events identified only in GS1, in both GS1 and GS2 and only in GS2 by PTM types. Only PTM events that can be localized to a specific residue were considered. Ac, acetylation; Ci, citrullination; Hy, hydroxylation; Me, methylation; Mt, methylthiolation; Ni, nitration; Ph, phosphorylation; Sn, S-nitrosylation. Figure 3: Dynamics of proteins and organism-specific PTM events between the two growth stages in the UBA and 5wayCG Leptospirilli . ( a ) The percentages of proteins and PTM events identified only in GS1 (green sections), in both GS1 and GS2 (orange sections), and only in GS2 (red sections). ( b ) The distribution of organism-specific PTM events identified only in GS1, in both GS1 and GS2 and only in GS2 by PTM types. Only PTM events that can be localized to a specific residue were considered. Ac, acetylation; Ci, citrullination; Hy, hydroxylation; Me, methylation; Mt, methylthiolation; Ni, nitration; Ph, phosphorylation; Sn, S-nitrosylation. 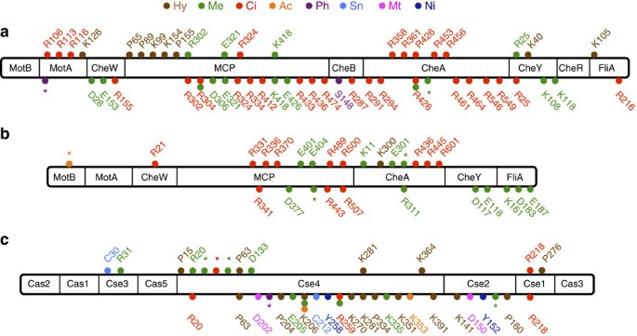Figure 4: Changes of PTM patterns from GS1 to GS2 in key pathways. (a) Chemotaxis gene cluster inLeptospirillumgroup II. (b) Chemotaxis gene cluster inLeptospirillumgroup III. (c) Cas gene cluster inLeptospirillumgroup II. Different PTM patterns were identified in the GS1 sample (above each bar) and the GS2 sample (below each bar). PTM events were colour-coded by PTM types and marked with amino acid types and residue positions. PTMs that cannot be localized to a specific residue were marked with an asterisk (*). Ac, acetylation; Ci, citrullination; Hy, hydroxylation; Me, methylation; Mt, methylthiolation; Ni, nitration; Ph, phosphorylation; Sn, S-nitrosylation. Full size image Figure 4: Changes of PTM patterns from GS1 to GS2 in key pathways. ( a ) Chemotaxis gene cluster in Leptospirillum group II. ( b ) Chemotaxis gene cluster in Leptospirillum group III. ( c ) Cas gene cluster in Leptospirillum group II. Different PTM patterns were identified in the GS1 sample (above each bar) and the GS2 sample (below each bar). PTM events were colour-coded by PTM types and marked with amino acid types and residue positions. PTMs that cannot be localized to a specific residue were marked with an asterisk (*). Ac, acetylation; Ci, citrullination; Hy, hydroxylation; Me, methylation; Mt, methylthiolation; Ni, nitration; Ph, phosphorylation; Sn, S-nitrosylation. Full size image The clustered regularly interspaced short palindromic repeats (CRISPRs) and associated proteins (Cas) provide bacteria and archaea with resistance to phage invasion [40] , [41] . The CRISPR/Cas locus of Leptospirillum group II is encoded on one recombined sequence block that is common across the genotypic series. Consistent with the calculated recent timing of this event [25] , the Cas proteins are identical among UBA, 5wayCG and other variants of Leptospirillum group II. Cas proteins showed very distinct PTM patterns between these two growth stages ( Fig. 4c ). Citrullination on Cse1 (CGL2_11386G0024 and UBAL2_8241G0432) was maintained across the two growth stages. Cse2 (CGL2_11386G0025 and UBAL2_8241G0431) was modified with four different types of PTMs only in GS2. PTMs on Cse3 (CGL2_11386G0028 and UBAL2_8241G0427) were only identified in GS1. Cse4 (CGL2_11386G0026 and UBAL2_8241G0430) was extensively modified in both GS1 and GS2, but PTMs clustered on distinct regions of the protein in the two different biofilm growth stages. The structures of Cse1, Cse2 and Cse3, predicted on the basis of homology modelling, suggest that the identified PTMs are localized on the surface residues of the structures ( Supplementary Fig. 3 , Supplementary Table 3 and Supplementary Data 4 ). Because of the semi-stochastic nature of MS/MS acquisition in shotgun proteomics, some low-abundance PTM events were identified with technical variability between individual runs. However, as each sample was measured after digestion using multiple proteases and in technical replicates, the identified PTM events aggregated across the six runs of a sample were reproducible and very few new PTM events were found with additional runs after the first three measurements ( Supplementary Fig. 4 ). Moreover, the percentage of organism-specific PTMs maintained between GS1 and GS2 was almost unchanged after the first two measurements as the PTM coverage increased. This indicates that the difference between aggregated PTM events identified in the two samples was not a result of run-to-run variability and the repeated measurements approached the detection limit of our methodology. Many modified peptides were identified along with their unmodified versions in a sample, which indicated partial modification of those peptides. The fractional occupancies of 3,287 and 3,207 unique PTM events were estimated in the GS1 and GS2 samples, respectively, with an average standard deviation of 6.5% ( Supplementary Fig. 5 and Supplementary Data 5 ). The reproducibility of these results was comparable to that of a previous study [28] . The quantified PTM events were separated into three ranges based on their fractional occupancy: low (<20%), medium (20–80%), and high (>80%), and the frequency of each range was compared for each type of PTM ( Fig. 5 ). The majority of PTM events had low fractional occupancy, which is in agreement with the fractional occupancy of phosphorylation from yeast [28] . However, most S-nitrosylation events had high fractional occupancy. The percentages of the PTM events in the low-occupancy range decreased from the GS1 to GS2 for all PTM types. 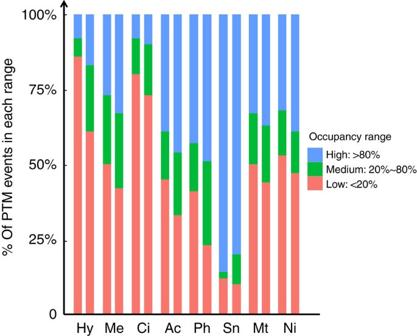Figure 5: Frequency of each fractional occupancy range for each type of PTM. PTM events in GS1 (left bars) and GS2 (right bars) were separated into three ranges: high occupancy of >80% (blue), medium occupancy of 20–80% (green), and low occupancy of <20% (red). Ac, acetylation; Ci, citrullination; Hy, hydroxylation; Me, methylation; Mt, methylthiolation; Ni, nitration; Ph, phosphorylation; Sn, S-nitrosylation. Figure 5: Frequency of each fractional occupancy range for each type of PTM. PTM events in GS1 (left bars) and GS2 (right bars) were separated into three ranges: high occupancy of >80% (blue), medium occupancy of 20–80% (green), and low occupancy of <20% (red). Ac, acetylation; Ci, citrullination; Hy, hydroxylation; Me, methylation; Mt, methylthiolation; Ni, nitration; Ph, phosphorylation; Sn, S-nitrosylation. Full size image Changes in PTM fractional occupancy were generally not correlated with changes in protein abundances, suggesting independent regulation of PTM abundances from protein abundances. For example, the fractional occupancy of the methylation at Glu35 of a pyruvate:ferredoxin oxidoreductase (UBAL3_7952G0038) from the Leptospirillum group III increased from 3% in the GS1 to 88% in the GS2 ( P -value=6.9 × 10 −4 , rank product test), but the protein abundance decreased by eightfold ( P -value=1.8 × 10 −2 , rank product test). Different PTM events on the same protein can also have different fractional occupancy changes. For example, the fractional occupancy of the citrullination at Arg113 of a 5wayCG-type chaperonin GroEL (CGL2_10776G0010) increased from 0.9% in GS1 to 9.6% in GS2 ( P -value=2.7 × 10 −2 , rank product test), but the fractional occupancy of the hydroxylation at Lys92 of the same protein decreased from 3.2 to 0.4% ( P -value=4.7 × 10 −2 , rank product test). PTM divergence between closely related co-existing bacteria Although the UBA and 5wayCG Leptospirilli share 95% average amino acid identity between their orthologues, we identified ~18,000 and ~25,000 organism-specific peptides that covered the positions with single amino acid polymorphisms (SAAPs) in GS1 and GS2, respectively. Amongst these organism-specific peptides, 1,373 and 1,457 PTM events were unambiguously assigned to the orthologues of specific organisms in GS1 and GS2, respectively. The conservation of PTM events between orthologues was analysed by mapping these organism-specific PTM events onto aligned orthologous sequences. Of those PTM events that can be localized to specific residues, only 30 and 21% of them were conserved in GS1 and GS2, respectively ( Fig. 6a ). The results were consistent between replicate measurements. 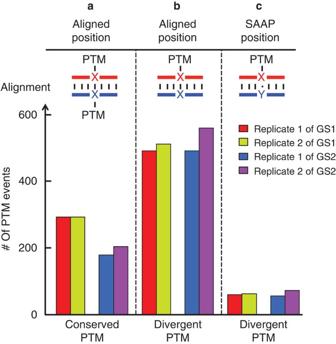Figure 6: Organism-specific PTM conservation and divergence between the UBA and 5wayCGLeptospirilliand their frequency. Orthologous proteins were aligned and PTMs were mapped to the modified residues. (a) PTM conservation at the aligned position with a conserved amino acid. (b) PTM divergence at the aligned position with a conserved amino acid. (c) PTM divergence at the position with SAAP. The bar graph shows the frequency of each case. X and Y represent an amino acid residue. Replicate 1 includes the first runs of the tryptic digest, the Lys-C digest and the Glu-C digest. Replicate 2 includes the second runs of the tryptic digest, the Lys-C digest and the Glu-C digest. Figure 6: Organism-specific PTM conservation and divergence between the UBA and 5wayCG Leptospirilli and their frequency. Orthologous proteins were aligned and PTMs were mapped to the modified residues. ( a ) PTM conservation at the aligned position with a conserved amino acid. ( b ) PTM divergence at the aligned position with a conserved amino acid. ( c ) PTM divergence at the position with SAAP. The bar graph shows the frequency of each case. X and Y represent an amino acid residue. Replicate 1 includes the first runs of the tryptic digest, the Lys-C digest and the Glu-C digest. Replicate 2 includes the second runs of the tryptic digest, the Lys-C digest and the Glu-C digest. Full size image Of these divergent PTM events, a total of 774 and 880 from the two replicates occurred on the aligned positions with a conserved amino acid between orthologous proteins of the UBA and 5wayCG Leptospirilli in GS1 and GS2, respectively ( Fig. 6b ). There were ~100 divergent PTM events that occurred on the SAAP position in a sample ( Fig. 6c ). Many SAAP events changed the amino acid type of a residue in one organism to another amino acid that cannot carry the same PTM in the other organism. As an example, the 815th residue of a transaldolase was an acetylated lysine in the 5wayCG-type orthologue (CGL2_11067G0037) but it was substituted by a glutamic acid that cannot be acetylated in the UBA-type orthologue (UBAL2_8692G0154) ( Supplementary Fig. 6A ). Some residues on the SAAP positions were modified with different PTMs. For example, there was a K267R substitution in a pair of orthologues annotated as ‘outer membrane efflux protein’, where the lysine of the 5wayCG-type orthologue (CGL2_11111G0096) was trimethylated, but the arginine of the UBA-type orthologue was citrullinated (UBAL2_8241G0570; Supplementary Fig. 6B ). The distribution of divergent and conserved PTMs and the distribution of PTM types by cluster of orthologous groups (COGs) are shown in Supplementary Figs 7 and 8 , respectively. COG enrichment of the divergent PTMs was compared between GS1 and GS2. Proteins with divergent PTMs were significantly enriched ( P -value <0.05, two-tailed Fisher’s exact test) in the COG categories of ‘Translation, ribosomal structure and biogenesis’ in GS1 and ‘Amino acid transport and metabolism’, ‘Replication, recombination and repair’, ‘Secondary metabolites biosynthesis, transport and catabolism’, and ‘Transcription’ in GS2. Conserved PTM events and divergent PTM events were compared in terms of fractional occupancy ( Supplementary Fig. 9 ). The majority of conserved PTM events and divergent PTM events belonged to the low fractional occupancy range, but significantly more divergent PTM events than the conserved PTM events were found in the high fractional occupancy range. This observation was consistent for both GS1 and GS2. Within the AMD biofilm, Leptospirillum group II likely uses the rTCA cycle for CO 2 fixation [39] . We identified every protein in the rTCA cycle from both UBA and 5wayCG Leptospirilli , with average sequence coverage of 82%. These proteins were extensively modified in both GS1 and GS2 samples. The PTM events were mapped onto the proteins’ predicted structures ( Fig. 7 and Supplementary Table 3 ). Most of the PTM events were localized on surface residues ( Fig. 7 and Supplementary Data 4 ). We focused on the organism-specific PTM events to study their dynamics between the two growth stages and divergence between organisms on the rTCA cycle ( Fig. 7 and Supplementary Fig. 10 ). There were PTM events that occurred only in a specific organism in one sample (for example, the PTMs on the fumarate reductase (GCL2_11068G0116 and UBAL2_7931G0249)) and PTM events that occurred across both organisms in both samples (for example, the hydroxylation at the P245 and citrullination at the R207 and R244 on the aconitate hydratase (CGL2_11068G0120 and UBAL2_7931G0253)). Some PTM events were specific to a growth stage and conserved across organisms (for example, the hydroxylation on the alpha subunit of succinyl-CoA synthetase (CGL2_11068G0122 and UBAL2_7931G0255) in GS1, Supplementary Fig. 10 ), whereas some PTM events were organism-specific in both samples (for example, a cluster of methylations at the D226, D227 and R232 on the UBA-type succinyl-CoA synthetase’s beta subunit (UBAL2_7931G0248)). 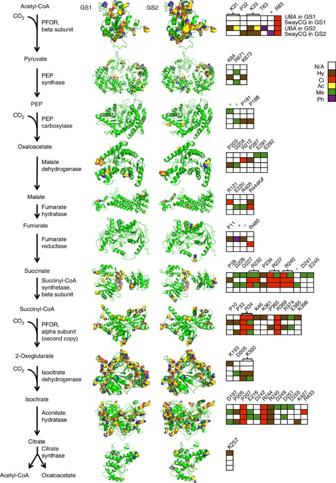Figure 7: Dynamics and organism-specific divergence of the PTM patterns in the rTCA cycle of theLeptospirillumgroup II. Modified residues that carried PTMs unique to theLeptospirillumgroup II (GS1 on the left and GS2 on the right) were highlighted with ball representation in the predicted structures (colour coding: green for backbone, yellow for carbon, blue for nitrogen, red for oxygen and orange for sulphur). For multi-subunit enzymes, only one subunit is shown here and the remaining inSupplementary Fig. 10. Residues with organism-specific PTMs were shown in grids marked with residue positions and colour-coded by PTM types. The four rows in each grid represent UBA-type ortholog in GS1, 5wayCG-type ortholog in GS1, UBA-type ortholog in GS2 and 5wayCG-type ortholog in GS2. PEP, phosphoenolpyruvate; PFOR, pyruvate:ferredoxin oxidoreductase. PTMs that cannot be localized to a specific residue were marked with an asterisk (*). Position with SAAP was marked with a number sign (#). Ac, acetylation; Ci, citrullination; Hy, hydroxylation; Me, methylation; Ph, phosphorylation. Figure 7: Dynamics and organism-specific divergence of the PTM patterns in the rTCA cycle of the Leptospirillum group II. Modified residues that carried PTMs unique to the Leptospirillum group II (GS1 on the left and GS2 on the right) were highlighted with ball representation in the predicted structures (colour coding: green for backbone, yellow for carbon, blue for nitrogen, red for oxygen and orange for sulphur). For multi-subunit enzymes, only one subunit is shown here and the remaining in Supplementary Fig. 10 . Residues with organism-specific PTMs were shown in grids marked with residue positions and colour-coded by PTM types. The four rows in each grid represent UBA-type ortholog in GS1, 5wayCG-type ortholog in GS1, UBA-type ortholog in GS2 and 5wayCG-type ortholog in GS2. PEP, phosphoenolpyruvate; PFOR, pyruvate:ferredoxin oxidoreductase. PTMs that cannot be localized to a specific residue were marked with an asterisk (*). Position with SAAP was marked with a number sign (#). Ac, acetylation; Ci, citrullination; Hy, hydroxylation; Me, methylation; Ph, phosphorylation. Full size image In this study, we optimized a shotgun proteomic approach for identification and quantification of a broad range of PTMs. Combining multiple proteases with the optimized HCD method significantly increased the sequence coverage of proteins, which allowed identification of more PTM events and estimation of their fractional occupancy. High-resolution MS/MS provided parts per million-level mass accuracy on every matched fragment ion of the identified peptides, which was essential for controlling the FDR of PTM identification. High-performance computing enabled searching an enormous sequence space with these many types of PTMs. In comparison with enrichment-based approaches, our new approach has the advantages of simultaneous detection of multiple types of PTMs and direct quantification of the fractional occupancy of PTM events. Furthermore, our approach only consumes micrograms of proteins, whereas the enrichment-based approaches typically require milligrams of proteins, which are not available for many environmental samples. Using this approach, we identified a large number of PTM events in laboratory-grown E. coli and in the dominant bacteria associated with two growth stages of a natural biofilm community in AMD. This model community has a well-curated protein database for effective database searching and the extensive prior work provided the ecological and evolutionary context for our results. PTM profiles of many proteins were substantially different between the two growth stages of the AMD community, indicating that dynamic PTMs may regulate the metabolic activities of organisms under different environmental conditions. Leptospirillum spp. are the primary producers in the AMD system, using the rTCA cycle for carbon fixation. Proteomic stable isotope probing has shown scant protein production and little net growth in GS2 biofilms, which suggests decreased carbon fixation [32] . However, we found no significant protein abundance changes for most enzymes in the rTCA cycle, as has been observed previously [38] . Particularly, the key carbon fixation enzyme, pyruvate:ferredoxin oxidoreductase, was highly abundant in both GS1 and GS2 (total spectral counts of 14,514 in GS1 and 11,160 in GS2). We believe the discrepancy between the expected decrease in rTCA cycle activity and the lack of corresponding protein abundance changes for rTCA enzymes can be explained by the PTM changes on these enzymes between the two growth stages ( Fig. 7 and Supplementary Fig. 10 ). We hypothesize that, in GS2, Leptospirillum group II bacteria may modulate the rTCA cycle activity through concerted PTM changes on the rTCA enzymes, while maintaining the protein stocks of these enzymes to be able to quickly respond to favourable conditions for growth and rapidly meet the demand for carbon fixation. This example shows the importance of taking PTM regulation into account when inferring the activity changes of enzymes from their abundance changes in microbial ecology studies. In the mature biofilms, Leptospirillum group II bacteria have been shown to increase the abundances of chemotaxis proteins in response to diminishing availability of nutrients [38] . Here we observed similar results, with a 3.7-fold increase in the protein abundance of MCP and 4.1-fold for CheA from GS1 to GS2. We additionally observed a number of PTM changes on chemotaxis-associated proteins that could alter environmental sensing and signal transduction ( Fig. 4a,b ). For example, a series of hydroxylations on MCP were observed only in GS1 within its predicted extracellular ligand-binding domain [42] . These changes could have profound effects on the ligand-binding activities and may generate distinct environmental sensory responses between the two growth stages. Methylation and demethylation of chemotaxis proteins is a well-known mechanism for regulating organisms’ mobility in response to different attractants and repellents [43] . Here, we observed a number of methylation events of the chemotaxis proteins that differ between the two growth stages. Overall, these results suggest that, during the ecological succession of the AMD biofilm, Leptospirillum group II bacteria not only increase protein abundances to achieve higher degree of mobility, but also may use PTM changes to alter their chemotaxis behaviours for environmental sensing. Viral defense is essential for natural communities. Here, the Cas proteins of Leptospirillum group II bacteria were highly abundant in both growth stages (total spectral counts of 3,008 in GS1 and 5,271 in GS2), but the Cas proteins were not detected in the E. coli laboratory culture. The abundances of Cas proteins may reflect the risk level of virus attack in the organisms’ environments, ranging from virtually none in the laboratory condition for E. coli , to medium risk in GS1 for Leptospirillum group II bacteria, and to high risk in GS2 with elevated stress and no significant growth. We believe the activity of the CRISPR/Cas system may also be regulated by dynamic PTMs ( Fig. 4c ) between the two growth stages to handle different levels or types of viral stresses. These PTMs were found to be located on the surface residues of proteins and, therefore, may exert regulatory effects by altering the protein–protein interactions or protein–nucleic acid interactions in the CRISPR/Cas complex. To the best of our knowledge, this is the first report of PTMs on the CRISPR/Cas system. The biotechnology applications of engineered Cas proteins need to consider potential structural changes and regulatory implications of PTMs [44] . The finding of extensive modifications in this study may provide the foundation for further biochemistry studies to determine the biological effects of PTMs in Cas proteins. Remarkable PTM divergence was found between the UBA and 5wayCG Leptospirilli . SAAPs between orthologous proteins in these organisms can directly contribute to PTM divergence on the SAAP position by substituting a modifiable residue with an unmodifiable residue. There was also a large portion of divergent PTMs that occurred in the vicinity of the SAAP positions. Such divergent PTMs could be caused by SAAPs on the motif that might alter modification enzyme–substrate interactions [45] . Because of regulatory roles of PTMs in protein activities, differential modifications may contribute to subtle functional variations between orthologous proteins and may have an important role in ecological and evolutionary divergence between closely related organisms. The dynamics and organism-specific divergence of PTMs may be interpreted using a trans / cis model adapted from gene regulation [17] . Changes in transcriptional factor ( trans -effects) or in regulatory DNA sequence ( cis -effects) could cause variations in gene expression between closely related organisms [46] . Similarly in protein post-translational modification, a modification enzyme ( trans -element) recognizes a motif on the protein ( cis -element) to carry out a modification reaction. The dynamics of PTMs between different conditions in the same organism is probably due to changes in the modification enzymes’ activities ( trans -effects). On the other hand, the divergence of PTMs between different organisms can be caused by polymorphism(s) on or around the target residue ( cis -effects) or a combination of cis -effects and trans -effects. Further study on model organisms will be needed to validate the cis- effects and trans- effects in the regulation of PTMs. In conclusion, our new proteomic approach revealed a broad range of PTMs on proteins from co-existing microorganisms in a natural biofilm community. The prevalence and variety of PTMs greatly expands the structural diversity and the functional promiscuity [44] of proteins. We believe dynamic PTMs are widely used in many ecological processes as a way of modulating enzyme activities in response to changes in environmental conditions. Closely related, but ecologically distinct, bacteria harboured notably divergent PTM patterns between orthologous proteins, which may contribute to their ecological divergence [24] . The findings of this study motivate further study of the role of PTMs in the ecology and evolution of microbial communities. Biofilm sampling and E. coli culture GS1 and GS2 biofilms were sampled at the AB Muck Dam site in the Richmond Mine at Iron Mountain, CA on 17 September 2010 (pH ~1, 39 °C). We used an E. coli cell culture from a previous study [47] . Briefly, the E. coli K-12 strain was cultivated aerobically with constant agitation (250 r.p.m.) at 37 °C in Luria-Bertani medium (pH 7.2). Cells were harvested when the culture reached an O.D. of ~0.8. Sample preparation The AMD biofilm samples and E. coli sample were prepared similarly. A total of 150 mg of biomass (wet weight) were lysed in 4% SDS (weight) dissolved in Tris buffer (100 mM, pH 8.0). Extracellular matrix of the biofilms was removed by centrifugation after the cell lysis. Extracted proteins were precipitated in 20% (volume) of trichloroacetic acid overnight at 4 °C and pelleted by centrifugation at 4 °C. Protein pellets were washed with ice-cold acetone three times and re-solubilized in guanidine (6 M) and dithiothreitol (10 mM). Bicinchoninic acid assays were conducted to estimate the protein concentration before adding dithiothreitol. Then, 50 μg of each sample was further processed with the filter-aided sample preparation method [48] , following the manufacturer’s protocol with minor modifications (Expedeon). Biofilm samples were digested with trypsin (Promega), Lys-C (Roche) and Glu-C (Roche) in parallel. E. coli sample was digested with trypsin and Lys-C in parallel. Each sample was first digested overnight in an enzyme:substrate ratio of 1:100 (weight:weight) at room temperature with gentle shaking, followed by a secondary digestion for 4 h. All digested peptide samples were stored at −80 °C. Two-dimensional LC-MS/MS measurements We used the multi-dimensional protein identification technology (MudPIT) [49] in our analytical workflow. In each MudPIT run, 25 μg of peptide from a biofilm sample or 10 μg of peptide from an E. coli sample was loaded offline into a 150-μm-I.D. two-dimensional back column (Polymicro Technologies) packed with 3 cm of C18 reverse phase (RP) resin (Luna, Phenomenex) and 3 cm of strong cation exchange (SCX) resin (Luna, Phenomenex). The back column loaded with peptides was de-salted offline with 100% Solvent A (95% H 2 O, 5% CH 3 CN and 0.1% formic acid) and washed with a 1-h gradient from 100% Solvent A to 100% Solvent B (30% H 2 O, 70% CH 3 CN and 0.1% formic acid) to move peptides from RP resin to SCX resin. Then, the back column was connected to a 100-μm-I.D. front column (New Objective) packed in-house with 15 cm of C18 RP resin and placed in-line with a U3000 quaternary HPLC pump (Dionex). Each MudPIT run was configured with 11 SCX fractionations using 5%, 7%, 10%, 12%, 15%, 17%, 20%, 25%, 35%, 50% and 100% of Solvent D (500 mM ammonium acetate dissolved in Solvent A). Each SCX fraction was separated by a 110-min RP gradient from 100% Solvent A to 60% Solvent B. The LC eluent was directly nanosprayed (Proxeon) into an LTQ Orbitrap Elite mass spectrometer (Thermo Scientific). Both MS scans and HCD MS/MS scans were acquired in Orbitrap with the resolution of 30,000 and 15,000, respectively. The top 10 most abundant precursor ions were selected for MS/MS analysis by HCD after each MS scan. Operational parameters critical for the optimum performance of the HCD MS/MS method included a minimum ion threshold of 1,000 to trigger MS/MS, normalized collisional energy of 30%, and the low m / z cutoff of 180 in MS/MS scans. In the CID MS/MS method, the top 20 most abundant precursor ions were selected for MS/MS analysis by CID after each MS scan and the fragment ion spectra were acquired with linear ion trap. Each proteolytic digest was measured in technical duplicates. Broad-range PTM searches with Sipros on Titan All Raw files were converted to FT1 and FT2 flat files using Raxport ( http://raxport.omicsbio.org ) and searched using Sipros ( http://sipros.omicsbio.org ). The E. coli runs were searched against the E. coli K-12 MG1566 genome database downloaded from NCBI in 2012 (the database is available as a FASTA file at the Chorus Project website, https://chorusproject.org/anonymous/download/experiment/3738367294184398156 ). A trypsin-digested GS2 AMD sample was first searched against the complete AMD database containing 79,633 proteins (available at the Chorus Project website, https://chorusproject.org/anonymous/download/experiment/264001236063703668 ), which were derived from ~80 billion base pairs of genomic information obtained from previous metagenomic characterizations of the Richmond Mine AMD system (NCBI BioProject accession code PRJNA20823 ). Based upon the preliminary search results, species that were not significantly detected in the sample were removed from the complete AMD database to reduce the sequence space. The final AMD database for PTM searches contained 15,523 proteins from seven organisms (available at the Chorus Project website, https://chorusproject.org/anonymous/download/experiment/-7500136186166692913 ), including Leptospirillum group II UBA, Leptospirillum group II 5wayCG, Leptospirillum group III, and four archaea [50] ( Ferroplasma I, G plasma, E plasma and A plasma). The broad-range PTM searches were conducted with Sipros 3.0 on a supercomputer, Titan, at Oak Ridge Leadership Computing Facility. All runs were searched with the following parameters: parent mass offsets of −1, 0, +1, +2, +3 Da; 0.03 Da and 0.01 Da of mass tolerances for parent ions and fragment ions, respectively; up to three missed cleavages; a maximum of two PTMs per peptides, and full enzyme specificity required. The following PTMs were dynamically searched: oxidation of methionine; hydroxylation of proline and lysine; deamidation of asparagine and glutamine; citrullination of arginine; monomethylation of arginine, lysine, aspartic acid and glutamic acid; dimethylation of arginine and lysine; trimethylation of lysine; phosphorylation of serine, threonine, tyrosine, histidine and aspartic acid; acetylation of lysine; S-nitrosylation of cysteine; nitration of tyrosine; methylthiolation of aspartic acid; and alkylation of cysteine by iodoacetamide. Oxidation and hydroxylation have an identical mass shift and so do deamidation and citrullination, but these isobaric PTMs modify different types of amino acid residues. A peptide that has residues modifiable by both types of isobaric PTMs was discarded, unless the mass shift can be localized to a specific residue with DeltaP >0 (described below) for the PSM. When a spectrum was matched to multiple peptides with the same highest score, Sipros ranked these peptides by their number of modifications. Unmodified peptides were ranked higher than modified peptides with a tied top score for a spectrum. Such ranking minimized the number of PTM identifications and allowed proper calculation of DeltaP scores (described below). A phosphorylated peptide candidate for a measured MS/MS spectrum was scored with three types of predicted MS/MS spectra to account for different neutral loss scenarios: (1) no neutral loss; (2) neutral loss of HPO 3 in the phosphorylated fragment ions; and (3) neutral loss of HPO 3 and H 2 O in the phosphorylated fragment ions. For the HCD and CID results shown in Supplementary Table 1 , the runs were searched with dynamic oxidation of methionine, dynamic deamidation of asparagine and glutamine and static alkylation of cysteine by iodoacetamide. The fragment ion mass tolerances for the CID run and HCD run were 0.5 Da and 0.01 Da, respectively. All the other search parameters were kept the same as mentioned above. Peptide filtering and protein inference The search result of each run was filtered individually to achieve 1% FDR at the peptide level estimated by concatenated reverse sequence identifications [34] . Proteins were inferred from the identified peptides using parsimony rules [51] . Briefly, indistinguishable proteins were combined into protein groups and subset proteins and subsumable proteins were removed. A minimum of two peptides, at least one of which must be unique, was required for each inferred protein or protein group. PTM localization We used Sipros to search a PTM on all modifiable residues in a peptide. Candidates with the same PTM on different positions of a peptide (PTM isoforms) were scored to identify the top-rank PSM for a spectrum. For a modified PSM, Sipros calculated the DeltaP score, which was the score difference between the top-rank modified peptide and its next lower-ranked PTM isoform [52] . For a modified PSM with a DeltaP >0, Sipros had information to localize the PTM on the top-rank peptide. For a modified PSM with a DeltaP=0, Sipros did not provide PTM localization, because the top two candidates with different modified residues cannot be differentiated by any fragment ions. Only modified peptides with localized PTMs (DeltaP >0) were used in the PTM dynamics and divergence analysis, except for noted examples in Figs 4 and 7 and Supplementary Fig. 10 . Database searching of synthetic phosphopeptide libraries We searched the first 20 libraries of the published study [35] . Each library’s MS/MS data were searched against its matched peptide database with concatenated reverse sequences and the result was filtered to achieve 1% FDR at the peptide level. The database searching and filtering parameters were kept the same as the broad-range PTM search, but only oxidation of methionine and phosphorylation of serine, threonine and tyrosine were dynamically searched. The identified phosphorylated spectra with DeltaP=0 were discarded, because the phosphorylation cannot be localized. Of the remaining modified spectra, 97% had correct PTM localization. Relative quantification of protein abundance All quantification was conducted with ProRata [53] ( http://prorata.omicsbio.org ). Briefly, ProRata re-constructed ion chromatograms for identified peptides using high mass accuracy (0.03 Da mass tolerance) and detected their chromatographic peaks. Both peak area and peak height were calculated for quantified peptides, but the peak height was used to represent the peptide abundance in this study due to its lower run-to-run variability. For protein quantification, ProRata summed peak heights of all quantified unique peptides from a protein and used the total peak height for protein relative abundance estimation. Quantification of PTM fractional occupancy ProRata calculated the total peak heights of all modified unique peptides that carried a specific PTM event and the total peak heights of both modified and unmodified unique peptides that covered the same residue. Fractional occupancy was calculated as the total peak height of a modified site out of the total peak height of this site. The fractional occupancy was 100% for the PTM sites that were not covered by any unmodified peptide. PTM divergence analysis Orthologous protein pairs between the UBA and 5wayCG Leptospirilli were obtained from our previous studies [24] , [54] . Sequence alignment was performed using EMBOSS Needle [55] ( http://www.ebi.ac.uk/Tools/psa/emboss_needle/ ). The PTM divergence analysis used the orthologous protein pairs satisfying the following requirements: both proteins in a pair must be identified; and at least one protein in a pair must have organism-specific localized PTMs. Statistical analysis Rank product test [56] was used to calculate the P -values for the changes of PTM fractional occupancy and the changes of protein abundances between GS1 and GS2. For the dynamic PTM and COG category enrichment analysis, P -values were calculated using a two-tailed Fisher’s exact test and corrected for multiple comparisons using the Benjamini–Hochberg method. Protein structure prediction MUFOLD [57] was used to predict the structures of Cas proteins and rTCA enzymes. UBA-type sequences of rTCA enzymes were used as the input for structure prediction. The top five structural templates in PDB were selected for each protein together with the optimal target-template alignment. The best model was then comprehensively determined by a composite score of the identity score, template coverage and model quality assessment scores. PyMOL ( http://www.pymol.org ) was then used to display the protein structures and mark the modified sites by ball structures. The solvent accessibility was calculated by DSSP [58] . The relative solvent accessibility was then obtained by dividing the maximum solvent accessibility in a fully exposed state for each residue [59] . A cutoff of 0.2 for relative solvent accessibility was used to determine the buried or exposed residues [60] . Raw files availability Mass spectrometric RAW files are available at the Chorus Project website: for E. coli ( https://chorusproject.org/anonymous/download/experiment/4c9bb6de186d43c3b9482c69beaea72c ) and for AMD microbial communities ( https://chorusproject.org/anonymous/download/experiment/e01b50f1e0d74765bd8438e0bade50a0 ). How to cite this article: Li, Z. et al. Diverse and divergent protein post-translational modifications in two growth stages of a natural microbial community. Nat. Commun. 5:4405 doi: 10.1038/ncomms5405 (2014).